Biological and physical controls in the Southern Ocean on past millennial-scale atmospheric CO2changes Millennial-scale climate changes during the last glacial period and deglaciation were accompanied by rapid changes in atmospheric CO 2 that remain unexplained. While the role of the Southern Ocean as a 'control valve' on ocean–atmosphere CO 2 exchange has been emphasized, the exact nature of this role, in particular the relative contributions of physical (for example, ocean dynamics and air–sea gas exchange) versus biological processes (for example, export productivity), remains poorly constrained. Here we combine reconstructions of bottom-water [O 2 ], export production and 14 C ventilation ages in the sub-Antarctic Atlantic, and show that atmospheric CO 2 pulses during the last glacial- and deglacial periods were consistently accompanied by decreases in the biological export of carbon and increases in deep-ocean ventilation via southern-sourced water masses. These findings demonstrate how the Southern Ocean's 'organic carbon pump' has exerted a tight control on atmospheric CO 2 , and thus global climate, specifically via a synergy of both physical and biological processes. The Southern Ocean is believed to play a key role in the global carbon cycle and millennial-scale variations in atmospheric CO 2 (CO 2,atm ), which in turn may amplify the impacts of longer-term external climate forcing on global climate [1] . This role stems from the unique control the Southern Ocean is thought to exert on ocean–atmosphere CO 2 exchange [1] , [2] , [3] by both facilitating the upward transport of nutrient- and CO 2 -rich water masses along outcropping density surfaces and their exposure to the atmosphere, and modulating the export of biologically fixed carbon into the ocean interior, where it is remineralized and may be effectively isolated from the atmosphere. It has been proposed that these two key aspects of the Southern Ocean’s role in the marine carbon cycle may have exerted a dominant control on past CO 2,atm change, for instance via variations of dust-driven biological carbon fixation in the sub-Antarctic [4] , the extent of circum-Antarctic sea ice [5] impeding effective air–sea gas equilibration [6] , and/or changes in the strength or position of southern hemisphere westerlies driving the residual overturning circulation in the Southern Ocean [7] , [8] . While all of these mechanisms for past CO 2,atm change are compelling, observational evidence that might constrain the extent to which they have operated, in particular the balance of biological versus physical (that is, air–sea gas exchange or ocean dynamical) impacts, remains ambiguous. In the sub-Antarctic Atlantic north of the Polar Front (PF), decreased biological export production, along with a diminished aeolian supply of dust (and by inference iron) to the surface ocean, has been found to parallel millennial-scale increases in CO 2,atm . These observations suggest a significant impact of dust-driven variations of the strength of the ‘organic carbon pump’ on CO 2,atm (refs 9 , 10 , 11 , 12 ). However, marked increases in CO 2,atm are also accompanied by enhanced export productivity south of the PF (ref. 7 ). Polar- and sub-polar Southern Ocean export productivity changes thus appear to have opposed each other, raising questions concerning the overall magnitude and sign of the impact of Southern Ocean ‘organic carbon pump’ on CO 2,atm , when integrated across both regions [11] , [13] . On the other hand, while 14 C evidence has provided direct support for a link between Southern Ocean carbon sequestration (and millennial-scale CO 2,atm variability) and physical/dynamical controls on air–sea CO 2 exchange [14] , these data remain sparse and only extend across the last deglaciation. Here we present sub-millennially resolved qualitative and quantitative proxy reconstructions of bottom-water [O 2 ] from sub-Antarctic Atlantic sediment core MD07-3076Q (14°13.7′W, 44°9.2′S, 3,770 m water depth; Fig. 1 ) to estimate the apparent oxygen utilization (AOU) in deep waters, which is closely (stoichiometrically) related to the amount of remineralized dissolved inorganic carbon (DIC) because of the consumption of oxygen during the degradation of organic carbon. We use two independent proxy approaches: first, we determined the redox-sensitive enrichment of uranium and manganese in authigenic foraminifer coatings [15] , and second, we measured the difference in carbon isotopic composition between pore waters at the zero-oxygen boundary and overlying bottom waters, which is assumed to be reflected in δ 13 C of the benthic foraminifer Globobulimina affinis and Cibicides kullenbergi , respectively (Δδ 13 C C. kullenbergi–G. affinis ; refs 16 , 17 ). Our deep sub-Antarctic Atlantic [O 2 ] reconstructions show a close correlation to CO 2,atm variations during the last deglacial- and glacial periods. The combination of our [O 2 ] reconstructions with analyses of 230 Th-normalized opal fluxes, an indicator of biological export production [7] , [18] , and deep water 14 C ventilation ages, along with a robust age model for our study core [14] , [19] , [20] (Methods), highlights that carbon sequestration changes in the southern high latitudes cannot be attributed solely to changes in local biological export production. Instead, they involve significant changes in Southern Ocean vertical mixing and air–sea gas exchange, having direct implications for millennial-scale CO 2,atm variations, since 65,000 years before present (BP). 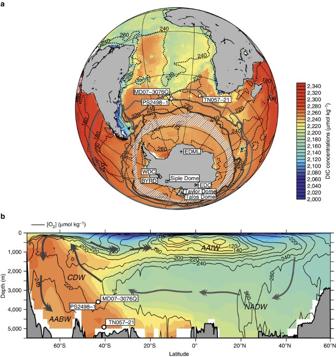Figure 1: Modern ocean DIC and oxygen concentrations. DIC levels (shaded) and [O2] (contours, in μmol kg−1)33,63in (a) Southern Ocean- and Atlantic Ocean bottom waters and (b) in a meridional transect across the Atlantic (averaged between 70°W and 20°E). Hatched area broadly represents the region, where the deep DIC reservoir directly ‘communicates’ with the surface ocean and the atmosphere along steep density surfaces (equivalent to the area of strong positive CO2fluxes across the air–sea interface in austral winter in the Southern Ocean64), which is unique in the global ocean today. White circles show study cores and open symbols mark the location of ice cores that document past changes in atmospheric CO2(CO2,atm; as inFigs 2and3). Thick lines show the modern positions of the PF, the sub-Antarctic Front (SAF) and the sub-Tropical Front (STF) (south to north)65. Arrows show general pathways of North Atlantic Deep Water (NADW), AABW (Antarctic Bottom Water), CDW (Circumpolar Deep Water) and Antarctic Intermediate Water (AAIW). Figure 1: Modern ocean DIC and oxygen concentrations. DIC levels (shaded) and [O 2 ] (contours, in μmol kg −1 ) [33] , [63] in ( a ) Southern Ocean- and Atlantic Ocean bottom waters and ( b ) in a meridional transect across the Atlantic (averaged between 70°W and 20°E). Hatched area broadly represents the region, where the deep DIC reservoir directly ‘communicates’ with the surface ocean and the atmosphere along steep density surfaces (equivalent to the area of strong positive CO 2 fluxes across the air–sea interface in austral winter in the Southern Ocean [64] ), which is unique in the global ocean today. White circles show study cores and open symbols mark the location of ice cores that document past changes in atmospheric CO 2 (CO 2,atm ; as in Figs 2 and 3 ). Thick lines show the modern positions of the PF, the sub-Antarctic Front (SAF) and the sub-Tropical Front (STF) (south to north) [65] . Arrows show general pathways of North Atlantic Deep Water (NADW), AABW (Antarctic Bottom Water), CDW (Circumpolar Deep Water) and Antarctic Intermediate Water (AAIW). Full size image Redox-sensitive U and Mn enrichment in foraminifer coatings The uranium to calcium ratio in authigenic (that is, in situ generated) coatings (c), proposed to vary with changes in sedimentary redox-conditions, and therefore with bottom-water [O 2 ] (ref. 15 ), has been measured on weakly chemically cleaned (‘host’) calcium carbonate (cc) shells (hereafter referred to as U/Ca cc+c ) of the planktonic foraminifer G. bulloides and the benthic foraminifer Uvigerina spp. (Methods). The uranium concentration in the authigenic coatings of foraminifera strongly exceeds the concentration in the foraminiferal shell matrix [21] , [22] . Thus, the overall U/Ca cc+c variability is marginally influenced by the uranium concentration in foraminifer shells, and has been proposed to primarily reflect coating-bound uranium variations instead that is inversely correlated with bottom-water oxygenation [15] . The co-variation of shell weights and U/Ca cc+c levels of G. bulloides , however, indicates that shell size and/or wall thickness variations may bias U/Ca cc+c ratios, via changes in the shell mass to surface-area ratio for example ( Supplementary Fig. 1 ). The normalization of coating-bound uranium levels to manganese concentrations circumvents this bias for two reasons: manganese has generally an opposing redox-behaviour to that of uranium [23] , [24] , [25] , and in particular manganese in weakly chemically cleaned foraminiferal tests mainly occurs in Fe-Mn-rich oxyhydroxides and/or Mn-rich carbonate overgrowths attached to the foraminiferal shell [22] , [26] , which may be supported by the observed co-variation of Fe/Ca cc+c and Mn/Ca cc+c levels of G. bulloides ( Supplementary Fig. 1 ). We propose that the U/Mn ratio of authigenic coatings in planktonic and benthic foraminifera, U/Mn c , serves as reliable indicator of redox-conditions in marine sediments independent of shell matrix variations. The close agreement of planktonic and benthic foraminifer U/Mn c suggests that it sensibly tracks early diagenetic redox-processes within the sediment consistent with previous findings [15] ( Supplementary Fig. 2 ). During the last glacial period, G. bulloides and Uvigerina spp. U/Mn c are both found to vary with changes in CO 2,atm ( Fig. 2 ). During the last deglaciation, the large early deglacial decrease in U/Mn c is clearly synchronous with the initial increase in CO 2,atm before 15 kyr BP, while the second pulse in U/Mn c in time with the CO 2,atm increase during the following Antarctic warming period (that is, the northern-hemisphere Younger Dryas period) is more equivocal ( Fig. 2 ). Our data are also in good agreement with changes in the authigenic enrichment of uranium in bulk sediments of Cape Basin core TN057-21 (ref. 27 ; location in Fig. 1 ), applying the most recent chronology of ref. 28 ( Fig. 2 ). This suggests a basin-wide relevance of observed changes in sedimentary redox-conditions in the central sub-Antarctic Atlantic for variations in CO 2,atm . 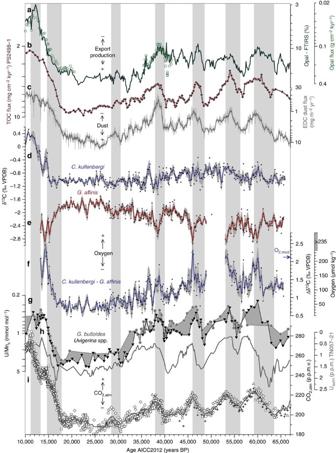Figure 2: Sub-Antarctic Atlantic bottom-water [O2] and productivity changes during the last deglacial and glacial periods. (a) Sedimentary opal content (line) and230Thorium-normalized opal fluxes (circles), (b) flux of TOC in PS2498-1 (ref.9; age scale adjusted as outlined in Methods), (c) Antarctic (EDC ice core) dust fluxes66, (d)C. kullenbergiδ13C (versus Vienna Pee Dee Belemnite (VPDB) standard), (e)G. affinisδ13C (versus VPDB), (f) Δδ13CC. kullenbergi–G. affinisand corresponding bottom-water [O2] (ref.16), arrow shows modern [O2] at the core site33, (g)G. bulloides(circles) andUvigerinaspp. (triangles) U/Mnc, (h) authigenic uranium concentrations in TN057-21 (ref.27,i) CO2,atmvariations recorded in the Antarctic ice cores BYRD (diamonds)67,68, EDML (crosses)47,69, EDC (right-pointed triangles)70, Siple Dome (squares)71, Talos Dome (triangles)47, Taylor Dome (circles)72and WDC (inverted triangles)73. All data refer to the AICC2012 age scale19,62. Lines ind–fshow 500 year-running averages with envelopes indicating the 500 year-window one-sigma standard deviation. Grey bars indicate periods of rising CO2,atm. Figure 2: Sub-Antarctic Atlantic bottom-water [O 2 ] and productivity changes during the last deglacial and glacial periods. ( a ) Sedimentary opal content (line) and 230 Thorium-normalized opal fluxes (circles), ( b ) flux of TOC in PS2498-1 (ref. 9 ; age scale adjusted as outlined in Methods), ( c ) Antarctic (EDC ice core) dust fluxes [66] , ( d ) C. kullenbergi δ 13 C (versus Vienna Pee Dee Belemnite (VPDB) standard), ( e ) G. affinis δ 13 C (versus VPDB), ( f ) Δδ 13 C C. kullenbergi – G. affinis and corresponding bottom-water [O 2 ] (ref. 16 ), arrow shows modern [O 2 ] at the core site [33] , ( g ) G. bulloides (circles) and Uvigerina spp. (triangles) U/Mn c , ( h ) authigenic uranium concentrations in TN057-21 (ref. 27 , i ) CO 2,atm variations recorded in the Antarctic ice cores BYRD (diamonds) [67] , [68] , EDML (crosses) [47] , [69] , EDC (right-pointed triangles) [70] , Siple Dome (squares) [71] , Talos Dome (triangles) [47] , Taylor Dome (circles) [72] and WDC (inverted triangles) [73] . All data refer to the AICC2012 age scale [19] , [62] . Lines in d – f show 500 year-running averages with envelopes indicating the 500 year-window one-sigma standard deviation. Grey bars indicate periods of rising CO 2,atm . Full size image Benthic foraminifer δ 13 C gradients and bottom-water [O 2 ] Redox-conditions in marine sediments generally reflect changes in organic carbon respiration within the sediment modulated by the downward diffusion of oxygen from bottom waters and/or the organic carbon supply to the sea floor [29] . Aerobic degradation of organic matter is the most efficient pathway of the respiration of organic carbon. Most of organic matter respiration therefore occurs above the sedimentary anoxic boundary. At the anoxic boundary, the diffusion of oxygen from the bottom water into the sediment is balanced by the rate of oxygen consumption during aerobic sedimentary organic carbon respiration in the sub-surface sediment column, such that [O 2 ] becomes zero. As organic carbon has typical δ 13 C values of about −22 ‰, the release of 13 C-depleted carbon during the degradation of organic matter substantially drives the δ 13 C gradient in marine sub-surface pore waters [30] . The total amount of aerobic sedimentary organic carbon respiration is thus a function of bottom-water [O 2 ] and is reflected in the δ 13 C difference between bottom waters and pore waters at the zero-oxygen boundary [16] , [30] . The deep infaunal foraminifer G. affinis actively chooses the low-oxygen microhabitat near or at the anoxic boundary within marine sub-surface sediments (in contrast to other benthic species) [31] . Assuming that C. kullenbergi δ 13 C reflects bottom-water δ 13 C (ref. 32 ), the offset of G. affinis δ 13 C from bottom water (that is, C. kullenbergi ) δ 13 C thus sensitively records the relative depletion of pore-water δ 13 C due to organic carbon respiraton [16] , [17] , [30] driven by the availability of oxygen in bottom waters. The occurrence of G. affinis in marine sediments may be in itself an indicator of an oxygen-limited sediment regime, where organic carbon is generally abundant and where the availability of oxygen is the main driver of organic matter respiration within the sediment [29] , because the characteristic zero-oxygen boundary in the shallow sub-surface of these sediments is the preferred habitat of G. affinis . The amount of pore water (that is, G. affinis ) δ 13 C depletion relative to bottom water (that is, C. kullenbergi ) δ 13 C is thus mostly insensitive to variations in organic carbon fluxes and scales instead with the amount of oxygen diffusing from the bottom water, allowing a quantification of bottom-water [O 2 ] (refs 16 , 17 ). In sediment core MD07-3076Q, G. affinis δ 13 C becomes markedly depleted by up to 1‰ relative to bottom-water ( C. kullenbergi ) δ 13 C during decreases in U/Mn c ( Fig. 2 ). The distinct negative offsets of G. affinis δ 13 C from C. kullenbergi δ 13 C mark millennial-scale increases in deep-water [O 2 ] (ref. 16 ) in the deep sub-Antarctic Atlantic that closely track rises in CO 2,atm during the last deglacial and glacial periods ( Fig. 2 ). According to the modern Δδ 13 C-[O 2 ] calibration of ref. 16 , bottom-water [O 2 ] in the deep sub-Antarctic Atlantic would have reached a minimum of about 40±20 μmol kg −1 during the peak glacial, which translates into a bottom-water [O 2 ] reduction of 175±20 μmol kg −1 from present-day levels of ∼ 215 μmol kg −1 at the core site [33] ( Fig. 2 ). During the last glacial period, that is, Marine Isotope Stage (MIS) 3, deep sub-Antarctic Atlantic [O 2 ] would have varied between 90±25 and 200±40 μmol kg −1 , in time with millennial-scale changes in CO 2,atm ( Fig. 2 ). Our quantification of deep sub-Antarctic Atlantic [O 2 ] relies on the assumption that bottom-water δ 13 C is reliably reflected in C. kullenbergi δ 13 C. This species has mostly been employed to reconstruct bottom-water δ 13 C in the southern high latitudes (because of the low abundance of other benthic epifaunal species); yet a difference of up to ∼ 0.6 ‰ has been observed between sparse glacial C. kullenbergi δ 13 C- and glacial C. wuellerstorfi δ 13 C measurements at ODP site 1090 in the Cape Basin [34] . This may imply that C. kullenbergi δ 13 C is anomalously depleted, for example, due to a slight infaunal habitat during glacial times [34] , and/or that δ 13 C measured on episodically occurring C. wuellerstorfi is anomalously enriched, for example, due to an affinity to anomalously well-ventilated water masses [35] and/or low carbon fluxes. If C. kullenbergi δ 13 C in MD07-3076Q does not adequately represent bottom-water δ 13 C at our core site, then absolute bottom-water [O 2 ] in the deep central sub-Antarctic Atlantic would be higher by up to ∼ 40 μmol kg −1 per 0.3‰-deviation of glacial bottom-water δ 13 C from glacial C. kullenbergi δ 13 C observed in MD07-3076Q ( Supplementary Fig. 3 ). However, our C. kullenbergi δ 13 C data are consistent with glacial benthic foraminifer ( C. kullenbergi and Cibicidoides spp.) δ 13 C measurements from different locations throughout the South Atlantic [34] , [36] , [37] , suggesting that they are representative of deep-water δ 13 C. Regardless of these quantitative uncertainties, the co-variation of the U/Mn c - and Δδ 13 C-based [O 2 ] reconstructions provides strong evidence for recurrent changes in deep sub-Antarctic oxygenation in parallel with CO 2,atm over the last glacial and deglacial periods. Changes in opal- and organic carbon fluxes The flux of biogenic silica (opal) to marine sediments in the southern high latitudes is assumed to reflect changes in organic carbon flux to the sea floor and in the export of organic carbon from the euphotic zone (that is, export production) [9] , [38] . Variations in the weight percentages of opal observed in MD07-3076Q are tightly correlated with 230 Th-normalized opal fluxes ( R 2 =0.94, P <0.05; Fig. 2 ; Supplementary Fig. 4 ), suggesting their accurate representation of past opal- (and therefore total organic carbon [9] , [38] ; TOC) fluxes in the sub-Antarctic Atlantic. This is supported by synchronous variations in the TOC flux observed in the neighbouring core PS2498-1 ( Fig. 2 , location in Fig. 1 ), which has been chronostratigraphically aligned to MD07-3076Q (Methods). As shown in Fig. 2 , opal- and TOC fluxes in the sub-Antarctic Atlantic show a close link to dust flux variations in Antarctic ice cores and changes in dust supply to the sub-Antarctic region [9] , which is consistent with earlier findings [9] , [10] . Estimates of radiocarbon ventilation ages Two metrics for deep-water ‘ventilation’ (that is, deep ocean versus atmosphere gas/isotope equilibration) that provide a measure of the average time since carbon in the ocean interior last equilibrated with the atmosphere are considered here: 14 C age offsets between coexisting benthic (B) and planktonic (Pl) foraminifera (B-Pl 14 C ventilation ages), and benthic 14 C age offsets from contemporary atmospheric 14 C ages (B-Atm 14 C ventilation ages). While the first provide an estimate of deep-ocean ventilation relative to the local mixed layer, the latter provide a direct estimate of deep-ocean ventilation relative to the contemporary atmosphere. As shown in Fig. 3 , B-Pl 14 C ventilation ages from sediment core MD07-3076Q broadly co-vary with changes in deep-ocean oxygenation (for example, with U/Mn c : R 2 =0.31, P <0.05) and CO 2,atm ( R 2 =0.43, P <0.05), both statistically significant within the 95% significance interval ( Supplementary Fig. 5 ). Parallel B-Atm 14 C ventilation age estimates agree with these observations, and confirm that B-Pl 14 C ventilation age fluctuations have not been significantly biased or masked by local surface-ocean radiocarbon disequilibrium effects (reservoir ages) ( Fig. 3 ). 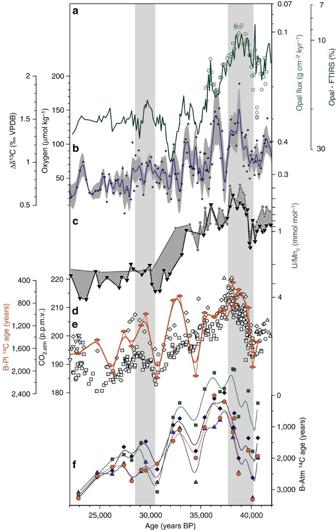Figure 3: Mid-glacial ventilation and carbon sequestration changes in the deep sub-Antarctic Atlantic. (a) Sedimentary opal content (line) and230Thorium-normalized opal fluxes (circles), (b) Δδ13CC. kullenbergi–G. affinisand corresponding bottom-water [O2] (ref.16,c)G. bulloides(circles) andUvigerinaspp. (triangles) U/Mnc, (d) Benthic-Planktonic (B-Pl)14C ventilation ages and the corresponding 1,000 years-running mean (thick line) plotted on top of (e) variations in CO2,atmrecorded in the Antarctic ice cores (open symbols, refs as inFig. 2), (f) benthic foraminifer14C age offset from atmospheric14C (Lake Suigetsu (green)74, Cariaco Basin (orange)75, Intcal09 (blue)76and Intcal13 (dark blue)77) shown as 1,000 years-running means (lines). Line and grey envelope inbshow a 500 year-running average and the 500 year-window one-sigma standard deviation, respectively. Grey bars indicate periods of rising CO2,atm. Figure 3: Mid-glacial ventilation and carbon sequestration changes in the deep sub-Antarctic Atlantic. ( a ) Sedimentary opal content (line) and 230 Thorium-normalized opal fluxes (circles), ( b ) Δδ 13 C C. kullenbergi – G. affinis and corresponding bottom-water [O 2 ] (ref. 16 , c ) G. bulloides (circles) and Uvigerina spp. (triangles) U/Mn c , ( d ) Benthic-Planktonic (B-Pl) 14 C ventilation ages and the corresponding 1,000 years-running mean (thick line) plotted on top of ( e ) variations in CO 2,atm recorded in the Antarctic ice cores (open symbols, refs as in Fig. 2 ), ( f ) benthic foraminifer 14 C age offset from atmospheric 14 C (Lake Suigetsu (green) [74] , Cariaco Basin (orange) [75] , Intcal09 (blue) [76] and Intcal13 (dark blue) [77] ) shown as 1,000 years-running means (lines). Line and grey envelope in b show a 500 year-running average and the 500 year-window one-sigma standard deviation, respectively. Grey bars indicate periods of rising CO 2,atm . Full size image These findings are consistent with similar analyses in the central deep sub-Antarctic Atlantic for the last deglaciation [14] . Although B-Pl 14 C ventilation age variations are more strongly influenced by surface-ocean reservoir age variations during the last deglaciation, decreasing B-Atm 14 C age offsets are linked to deglacial increases in CO 2,atm , in particular during the early deglacial period [14] . Notably, absolute foraminifer 14 C ages appear to be slightly too young during the mid-glacial period, perhaps due to uncertainties associated with background corrections, which are especially important for old (>30 kyr BP) sample material. In practice, these background corrections are based on one radiocarbon-dead spar calcite sample measured in each sample batch (that is, an accelerator mass spectrometry (AMS) sample carousel), whose apparent radiocarbon content is subtracted from the measured radiocarbon content of all the foraminifer samples measured in that sample carousel. If the true background deviates from the measured background in this single sample, then B-Atm 14 C and Pl-Atm 14 C age offsets may deviate significantly from their true absolute values. Godwin Radiocarbon Laboratory-internal backgrounds compiled for the 4 years from April 2011 to January 2015 amount to 14 C/ 12 C 0 =5.3±1.5 × 10 −15 ( Supplementary Fig. 6 ). Considering a one-off estimate of the background that is slightly smaller (that is, 14 C/ 12 C 0 =4 × 10 −15 ; within 1 s.d. of the mean) or larger (that is, 14 C/ 12 C 0 =6 × 10 −15 ; within 1 s.d. of the mean), this would result in B-Atm 14 C and Pl-Atm 14 C age offsets that are shifted towards slightly lower and higher absolute values respectively, without affecting the overall variability in each time-series ( Supplementary Fig. 7 ). As benthic and planktonic 14 C ages have been obtained from the same AMS sample carousels in this study, B-Pl 14 C ventilation ages are not affected by these uncertainties and are essentially the same irrespective of the applied background correction ( Supplementary Fig. 7 ). Therefore, while our absolute B-Atm 14 C and Pl-Atm 14 C age offsets are dependent on the accuracy of our background corrections (which are arguably difficult to assess), relative changes in B-Atm 14 C ventilation ages and absolute variations in B-Pl 14 C ventilation ages remain robust. As shown in Fig. 3 , these clearly co-vary with our estimates of bottom-water oxygenation in the deep sub-Antarctic Atlantic (see also Supplementary Fig. 5 ). Changes in the elemental composition of foraminifer coatings and bottom-water versus pore-water δ 13 C gradients, as described above, demonstrate that the amount of remineralized carbon sequestered in the deep sub-Antarctic Atlantic has varied substantially and inversely with respect to millennial-scale CO 2,atm changes ( Fig. 2 ). These observations confirm a role for the Southern Ocean ‘organic carbon pump’ in regulating CO 2,atm (refs 3 , 10 , 11 ). Below, we assess the quantitative impact of the inferred ‘biological carbon pump’ changes on CO 2,atm , as well as their governing biological and/or physical/dynamical controls. Bottom-water [O 2 ] reconstructions at our core site via Δδ 13 C C. kullenbergi – G. affinis provide the basis for a quantification of the amount of respired carbon in the deep sub-Antarctic Atlantic [16] , [30] , provided the modern Δδ 13 C-[O 2 ] relationship holds for the past. In principle, seawater [O 2 ] consists of a saturated [O 2 ] component ([O 2 ] sat ) arising from the solubility-controlled O 2 exchange between the atmosphere and the surface ocean, a biological [O 2 ] component associated with the release and drawdown of [O 2 ] during photosynthesis and respiration ([O 2 ] bio ), and a preformed disequilibrium [O 2 ] component ([O 2 ] diseq ) due to inefficiencies in air–sea gas exchange ([O 2 ] insitu =[O 2 ] sat +[O 2 ] bio +[O 2 ] diseq ) [39] . Assuming that ocean [O 2 ] is in equilibrium with the atmosphere ([O 2 ] diseq ∼ 0) and that last glacial ocean [O 2 ] sat was slightly higher than today ([O 2 ] sat,modern =345 μmol kg −1 ) mostly due to a decrease in ocean temperature ([O 2 ] sat,glacial =360 μmol kg −1 ; Methods), the amount of [O 2 ] depletion at ocean depth (AOU=−[O 2 ] bio =[O 2 ] sat −[O 2 ] insitu ) should scale with the formation of respired carbon according to a constant stoichiometric Redfield ratio of C:[O 2 ]=117:−170 (ref. 40 ). Changes in bottom-water [O 2 ] (and AOU) in the sub-Antarctic Atlantic would therefore provide a direct quantitative measure of the amount of carbon sequestered in the southern high-latitude ocean, and thus the efficiency of the biological ‘organic carbon pump’ [16] . Converting our AOU estimates into respired carbon concentrations (AOU Holocene =(345−215) μmol kg −1 , (AOU MIS2 =(360−40)±20 μmol kg −1 , ΔAOU Deglaciation =190±20 μmol kg −1 )based on the Redfield ratio of C:[O 2 ]=117:−170 (ref. 40 ) gives a respired DIC contribution of 220±14 μmol kg −1 to the total DIC pool at the core site during the last glacial maximum (LGM). This is higher by 130±14 μmol kg −1 compared with the Holocene [33] , indicating greater respired carbon accumulation during the LGM. During millennial-scale variations in CO 2,atm during the last glacial, respired carbon levels varied by 75±28 μmol kg −1 between 110±28 μmol kg −1 (during peak CO 2,atm levels) and 185±14 μmol kg −1 (during minimum CO 2,atm levels) assuming that [O 2 ] sat was not significantly different from LGM levels (that is, AOU MIS3‘CO 2 max' =(360−200)±40 μmol kg −1 , AOU MIS3‘CO 2 min' =(360−90)±25 μmol kg −1 , ΔAOU MIS3 =110±40 μmol kg −1 ). If we assume that the respired carbon lost from the deep sub-Antarctic Atlantic, where it was sequestered away from the atmosphere was transferred to a non-respired marine carbon pool that in turn equilibrated with the atmosphere via a surface-ocean DIC ‘buffer factor’ (that is, Revelle factor) of ∼ 10 (ref. 41 ; Methods), our AOU and respired carbon estimates from the deep sub-Antarctic may only explain the full amplitude of observed CO 2,atm , if they are representative of a significant fraction of the global deep ocean, that is, at least ∼ 33% during the mid-glacial period and ∼ 45% during the early deglaciation (Methods). This would roughly correspond to the deep ocean below 2.9 and 2.3 km, respectively (Methods). These depths broadly agree with the depth of the putative glacial ‘chemical divide’ ( ∼ 3 km water depth in the Atlantic) [42] , and are supported by qualitative proxy data showing a decrease in oxygenation and radiocarbon ventilation in the global ocean below 2 km during the last peak glacial period [43] , [44] . The smaller the volume of the global deep ocean that experienced similar changes in AOU and respired carbon to our sub-Antarctic Atlantic site, the smaller the likely oceanic impact on CO 2,atm concentrations. Our calculations have two major caveats. First, we ignore possible open-system effects due to the interaction of deep waters with sediments, and second, we may have underestimated glacial deep sub-Antarctic Atlantic [O 2 ], in the case that deep sub-Antarctic Atlantic C. kullenbergi δ 13 C values are strongly negatively biased versus bottom-water δ 13 C. Any open-system effects involving a degree of ‘carbonate compensation’ (on multi-millennial timescales) would tend to enhance the impact of marine respired carbon inventory changes on CO 2,atm (Methods). If true glacial bottom-water [O 2 ] were higher than estimated in MD07-3076Q for instance via an anomalous depletion of C. kullenbergi δ 13 C from bottom-water δ 13 C by 0.3‰, as mentioned above, deglacial changes in respired carbon and AOU (and thus the oceanic impact on CO 2,atm ) would be reduced by ∼ 20%, as LGM AOU values would be lower ( Supplementary Fig. 3 ). In contrast, our estimates of respired carbon changes during the last mid-glacial period remain to a large extent similar as they are based on relative [O 2 ] changes ( Supplementary Fig. 3 ). Our calculations are rough estimates that are intended only to provide a first indication of the potential impact of our observed marine carbon sequestration changes on CO 2,atm . To determine the full impact of changes in deep-ocean respired carbon levels on CO 2,atm concentrations, our estimates would need to be corroborated by further reconstructions of past bottom-water oxygen- and DIC concentrations from throughout the global ocean, in particular in the volumetrically most significant Pacific Ocean. The analysis above demonstrates the potential quantitative significance of the oxygenation changes that we observe, and more specifically of the role of the Southern Ocean ‘organic carbon pump’ in regulating CO 2,atm (refs 3 , 10 , 11 ). However, it remains to be shown whether the observed decreases in ‘organic carbon pump’ efficiency resulted primarily from decreases in export productivity (allowing oxygen to increase due to reduced organic carbon remineralization in the ocean interior) or primarily from increases in ocean ‘ventilation’ (causing carbon loss to the atmosphere with direct oxygen gain of the ocean interior). Below, we address this question by reference to our export productivity- and 14 C ventilation age estimates. The observed correlation between changes in the dust supply to the southern high-latitude regions and in export production in the central sub-Antarctic Atlantic (as recorded by variations in opal- and TOC fluxes [9] ; Fig. 2 ) supports earlier findings of a dust-driven biological organic carbon pump in the sub-Antarctic Atlantic [9] , [10] . The close relationship between variations in sub-Antarctic export production and CO 2,atm changes ( Fig. 2 ) would be consistent with a significant impact of the efficiency of the sub-Antarctic biological organic carbon pump on surface-ocean DIC levels, and thus on CO 2,atm (refs 9 , 10 , 11 ). The correlation between opal- and TOC fluxes and bottom-water [O 2 ] in the sub-Antarctic Atlantic ( Fig. 2 ) may point to a role of organic carbon respiration at depth driving deep sub-Antarctic Atlantic bottom-water oxygenation. To test whether export production was the major driver of our observed deep-ocean [O 2 ] changes (and therefore of the associated changes in deep-ocean respired carbon sequestration), we make use of the unique microhabitat of G. affinis near the anoxic boundary in marine sediments and the associated mechanisms that drive its δ 13 C signature. Notably, negative excursions of G. affinis δ 13 C are observed during each of the marked CO 2,atm rises during MIS 3 and the last deglaciation. These excursions indicate that total organic carbon respiration within deep sub-Antarctic Atlantic sediments increased at times of reduced opal- and TOC fluxes, that is, reduced export production ( Fig. 2 ). An increase in sedimentary organic carbon respiration (that is, pore water/ G. affinis δ 13 C depletions) would be driven by an increase in organic carbon flux, an increase in bottom-water [O 2 ], or both of these together. As the first is evidently not the case ( Fig. 2 ), we conclude that sedimentary carbon respiration must have instead been driven by enhanced deep-ocean ‘ventilation’ (that is, circulation/ convection rates and/or air–sea gas exchange) supplying oxygen to the deep sub-Antarctic Atlantic. Alternatively, a decreased oxygen demand in bottom waters due to diminished organic carbon fluxes and less respiration of organic matter in a benthic ‘fluff’ layer could facilitate the diffusion of oxygen into the sediment, and drive the G. affinis δ 13 C signal more negative. However, a poor inverse correlation between epibenthic and deep infaunal benthic foraminifer δ 13 C over past millennial timescales ( Fig. 2 ; R 2 =0.0001, N =258, Supplementary Fig. 8 ) would appear to rule out this scenario. We therefore conclude that the observed changes in ‘organic carbon pump’ efficiency and deep sub-Antarctic carbon storage were not only controlled by changes in export productivity but must also have involved biology-independent processes that contributed to past CO 2,atm changes specifically by enhancing ocean–atmosphere CO 2 exchange in the Antarctic region ( Fig. 2 ). Our interpretation is confirmed by parallel estimates of deep-water 14 C ‘ventilation ages’ ( Fig. 3 ). We observe that the marked CO 2,atm rise around 38 kyr BP is paralleled by a decrease in B-Atm 14 C ventilation ages of ∼ 2,000 14 C years. A consistent link between deep-ocean (B-Atm and B-Pl) 14 C ventilation and CO 2,atm variability is further supported by a high and statistically significant correlation coefficient between them (up to R 2 =0.6, P <0.05; Supplementary Fig. 5 ). The good correlation between (B-Atm and B-Pl) 14 C ventilation ages, deep-water [O 2 ] and CO 2,atm provides strong independent support for changes in the air–sea equilibration of deep waters in the Southern Ocean and their link to changes in respired carbon storage. It has previously been shown that the incursion of well-ventilated northern-sourced waters into the sub-Antarctic Atlantic was reduced during intervals of rising CO 2,atm (refs 20 , 28 ). On this basis, the periods of increased 14 C ventilation that we observe would therefore specifically reflect periods of increased local dominance of southern-sourced deep waters and an ‘improvement’ of their ventilation state. Numerous processes have been suggested to have caused changes in vertical mixing in the southern high latitudes, including for instance the intensity and/or the position of the southern hemisphere westerlies [7] , [8] , a retreat of circum-Antarctic sea ice [6] , a decline in the formation and advection of northern component waters [45] and/or changes in surface buoyancy fluxes [46] . It remains currently impossible to evaluate the relative importance of these specific processes and their controls on CO 2,atm . Nevertheless, the strong co-variations of our abyssal oxygenation and ventilation proxies with CO 2,atm confirm that some combination of dynamical (that is, residual circulation and shallow mixing) and/or physical (gas exchange efficiency) processes in the southern high-latitude region indeed had a significant impact on deep-ocean carbon sequestration [3] , [7] , [19] , [45] , [47] ( Fig. 4 ). 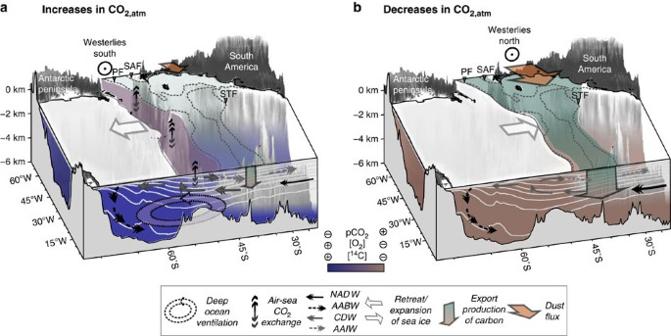Figure 4: Schematic view on the southern high-latitude Atlantic during millennial-scale CO2,atmvariations based on new and existing proxy evidence. (a) Dust-driven decreases of export production in the sub-Antarctic Atlantic9,10during the last glacial and deglacial periods were accompanied by decreases in deep carbon storage in the Southern Ocean (this study and ref.48). The latter was further promoted by increases in the air-sea CO2exchange south of the PF and in the ventilation of the deep carbon pool (this study and ref.48), causing millennial-scale increases in CO2,atm, as postulated earlier3,7. (b) Enhanced dust-driven, biological export of carbon to the deep sub-Antarctic Atlantic9,10paralleled increases in deep Southern Ocean respired carbon levels during the last glacial period and the last deglaciation (this study and ref.48). The enhanced Southern Ocean carbon pool was effectively isolated from the atmosphere by decreases in air–sea CO2equilibration in the Antarctic region and a poor 'ventilation' of the deep-ocean during these times (this study and ref.48), leading to decreases in CO2,atmduring the last 70,000 years, as proposed previously3,7. Accompanying changes in sea ice5,6and the westerly position/strength7,8are debated and remain speculative. The modern positions of ocean fronts (as inFig. 1) and ocean density surfaces (white lines) are shown as reference. Figure 4: Schematic view on the southern high-latitude Atlantic during millennial-scale CO 2,atm variations based on new and existing proxy evidence. ( a ) Dust-driven decreases of export production in the sub-Antarctic Atlantic [9] , [10] during the last glacial and deglacial periods were accompanied by decreases in deep carbon storage in the Southern Ocean (this study and ref. 48 ). The latter was further promoted by increases in the air-sea CO 2 exchange south of the PF and in the ventilation of the deep carbon pool (this study and ref. 48 ), causing millennial-scale increases in CO 2,atm , as postulated earlier [3] , [7] . ( b ) Enhanced dust-driven, biological export of carbon to the deep sub-Antarctic Atlantic [9] , [10] paralleled increases in deep Southern Ocean respired carbon levels during the last glacial period and the last deglaciation (this study and ref. 48 ). The enhanced Southern Ocean carbon pool was effectively isolated from the atmosphere by decreases in air–sea CO 2 equilibration in the Antarctic region and a poor 'ventilation' of the deep-ocean during these times (this study and ref. 48 ), leading to decreases in CO 2,atm during the last 70,000 years, as proposed previously [3] , [7] . Accompanying changes in sea ice [5] , [6] and the westerly position/strength [7] , [8] are debated and remain speculative. The modern positions of ocean fronts (as in Fig. 1 ) and ocean density surfaces (white lines) are shown as reference. Full size image Furthermore, our findings are entirely consistent with recently published sedimentary redox-sensitive trace element data from the Antarctic Zone of the Atlantic Ocean [48] . These data show that the accumulation of authigenic uranium (and therefore oxygenation) in the Antarctic Atlantic is generally inversely correlated with opal fluxes (that is, organic carbon fluxes) over the past 80,000 years, ruling out a dominant control of local surface-ocean productivity on deep Antarctic Atlantic [O 2 ] and deep-ocean respired carbon levels south of the PF (ref. 48 ). The combination of our sub-Antarctic study with the Antarctic study of ref. 48 provides strong evidence for millennial-scale changes in the respired carbon concentrations across the entire deep high-latitude South Atlantic, varying in parallel with CO 2,atm during the last glacial period and deglaciation, and for a significant impact of physical ‘ventilation’ processes (that is, overturning circulation, mixing and/or air–sea gas exchange) on changes in deep-ocean respired carbon sequestration and millennial-scale CO 2,atm in the past. In conclusion, our results show that pulses of CO 2,atm during the last glacial- and deglacial periods coincided with increases in the ventilation of the southern high-latitude deep ocean (specifically via regions of deep-water formation in the Southern Ocean [7] , [48] ), in addition to reductions in sub-Antarctic export productivity. By ruling in a role for variations in both the strength and the efficiency of the biological carbon pump via changes in the biological carbon export as well as the air–sea CO 2 exchange and Southern Ocean vertical mixing, the findings reconcile two opposing theories for the Southern Ocean’s role in past millennial-scale CO 2,atm variability [3] , [7] , [10] , [11] , [12] , [47] . Further work, for example using numerical model simulations will be required to quantify more precisely the contributions of (sub-polar zone) biological export productivity changes and (polar zone) physical/dynamical changes to deep-ocean carbon sequestration, as well as their down-stream effects on low-latitude export production [49] . Nevertheless, our data emphasize that while biological carbon export to the deep ocean is ultimately what permits ocean dynamics and air–sea exchange to impact on CO 2,atm by continually tending to ‘recharge’ the abyssal carbon pool, the rate of equilibration of the deep ocean with the atmosphere will ultimately determine whether or not the biological ‘organic carbon pump’ is efficient or not at sequestering CO 2 ( Fig. 4 ). Thus, ocean physics and marine biology acted together, synergistically, to repeatedly nudge the Southern Ocean from carbon sink to carbon source, with a direct impact on global climate over the last ∼ 65,000 years. Regional setting and chronology Sediment core MD07-3076Q (14°13.7′W, 44°9.2′S, 3,770 m water depth) is bathed in Lower Circumpolar Deep Water, which is formed by the entrainment of northward spreading DIC- and preformed nutrient-rich Circumpolar Deep Water into southward flowing DIC-low and regenerated nutrient-rich North Atlantic Deep Water [50] . Chronological control of sediment core MD07-3076Q is based on 14 C measurements of mono-specific planktonic foraminifer samples, which have been adjusted for variations in surface-ocean reservoir ages [14] . The 14 C-based age constraints are complemented by the stratigraphic alignment of abundance variations of the cold-water species Neogloboquadrina pachyderma (sinistral-coiling) with rate changes in Antarctic temperature over time [19] . Age model uncertainties, mainly a function of age marker density, amount to 1,600±500 years during the last glacial period and to 1,200±400 years after 27 kyr BP (ref. 19 ). Resulting sedimentation rates range between 5 cm kyr −1 during the last deglaciation and 15 cm kyr −1 during MIS 3. Element composition of authigenic foraminifer coatings Down-core measurements of U/Ca cc+c and U/Mn c have been made on 18–25 specimens of the planktonic foraminifer G. bulloides (250-300 μm size fraction) and the 5–13 specimens of the benthic infaunal foraminifer Uvigerina spp. (250-300 μm size fraction). Foraminifera have been weakly chemically cleaned (clay removal and silicate picking) to maintain foraminiferal coatings but to remove extraneous detritus [15] . Cleaned foraminifera have been dissolved in 0.1 M nitric acid for inductively coupled plasma (ICP)-atomic emission spectroscopy analyses. The samples were subsequently re-diluted to 10 p.p.m. Ca 2+ concentration and elemental concentrations have been determined by ICP-mass spectrometry [15] . Mean s.d. of U/Mn c of six duplicate samples is 0.08±0.06 mmol mol −1 . Given the high sedimentation rates of 15 cm kyr −1 , the impact of potential sedimentary re-oxidation processes (‘burn-down’ effects) of already precipitated uranium complexes is negligible for the interpretation of U/Ca cc+c and U/Mn c ratios. Reconstruction of bottom- to pore-water δ 13 C gradients Stable isotopic analyses on G. affinis and C. kullenbergi have been performed on 1–4 specimens (>150 μm size fraction) on Finnigan Δ+ and Elementar Isoprime mass spectrometers. The results are reported with reference to the international Vienna Pee Dee Belemnite (VPDB) standard. VPDB is defined with respect to the NBS-19 calcite standard. The mean external reproducibility of carbonate standards is σ±0.03 ‰. In MD07-3076Q, Δδ 13 C C. kullenbergi–G. affinis has been determined from δ 13 C measurements of benthic foraminifera from the same sediment sample, and has been converted into bottom-water [O 2 ] after ref. 16 . The calibration error associated with bottom-water [O 2 ] reconstructions using this method is ±17 μmol kg −1 (ref. 16 ). Analytical uncertainties of benthic δ 13 C analyses (two-sigma) translate into a bottom-water [O 2 ] uncertainty of ±8 μmol kg −1 . We have smoothed our high-resolution record by a running 500 year-window (solid line in Fig. 2 ) to reduce such biases and those from intra-specific δ 13 C variations. Mean bottom-water [O 2 ] have been determined for the LGM (23-18 kyr BP) as well as CO 2 minima (40.2-39.9 kyr BP, 48.4-47.6 kyr BP, 56.7-55.7 kyr BP, 63.6-63.0 kyr BP) and -maxima (38.8-38.0 kyr BP, 46.3-45.8 kyr BP, 53.6-53.3 kyr BP and 59.3-58.8 kyr BP) during MIS 3. Errors reported in our study are one-sigma standard deviations of our bottom-water [O 2 ] estimates during these periods. Calculation of deep-ocean and atmospheric carbon budgets [O 2 ] saturation levels are calculated according to ref. 51 assuming a glacial increase in salinity from present-day ( ∼ 35 p.s.u.) by ∼ 2 p.s.u. and a decrease in deep-ocean temperatures from modern-day values ( ∼ 1 °C) by 2 °C in the deep Southern Ocean [52] . [O 2 ] saturation in the glacial deep Southern Ocean increased by ∼ 15 μmol kg −1 from modern-day levels ( ∼ 345 μmol kg −1 ) (ref. 33 ). To estimate the amount of carbon that is transferred to the atmosphere from the ocean’s remineralized carbon pool (sequestered in the deep ocean), via the ocean’s non-remineralized carbon pool (in equilibrium with the atmosphere), we adopt the conceptual framework of ref. 41 , whereby: Here, Δ c soft and Δ c carb are DIC changes for the ocean’s total remineralized carbon pool (that is not in equilibrium with the atmosphere), due to changes in the soft-tissue pump and the carbonate pump (for instance via changes in the export of organic carbon and carbonate to the ocean interior), respectively. Our estimate of Δ c DIC during the last deglacial increase in CO 2,atm (Δ c DIC =130±14 μmol kg −1 ) and during mid-glacial CO 2,atm changes (Δ c DIC =75±28 μmol kg −1 ) determined above from oxygenation estimates provides an estimate of Δ c soft , during these time intervals, and we assume that the associated Δ c soft is approximately three times smaller (for example, as observed spatially in the modern ocean) [41] , yielding: where is the whole-ocean average change in remineralized carbon during the investigated time intervals. It is given by the product of the change observed at our core location and the fraction ( f ) of the total ocean volume that also experienced this magnitude of change: Assuming that the rest of the ocean volume experienced no significant change in respired DIC, remaining well-equilibrated with the atmosphere, the fraction of the ocean f , and therefore the deep-ocean volume V d and the upper ‘boundary’ of the deep-ocean z' , may be calculated that would account for the last early deglacial and mid-glacial atmospheric pCO 2 changes of ∼ 50 and ∼ 20 p.p.m. (for glacial background pCO 2 levels of 190–200 p.p.m. ), if affected by similar changes in AOU and respired DIC levels as our sub-Antarctic Atlantic core site. We have calculated the deep-ocean volume V d and z' based on the GEBCO bathymetric data set (excluding the Arctic Ocean) archived by the British Oceanographic Data Centre (http://www.gebco.net/), according to: that is the sum of all volumes of grid boxes (distance in west-east direction (km) times distance north-south direction (km) times depth), where φ is latitude, λ is longitude, Δ φ and Δ λ represent the grid spacing of the bathymetric data set, r is the Earth's radius, z the water depth and z' the upper limit of the deep ocean. Opal measurements Opal concentrations were measured on ∼ 400 samples by means of Fourier transform infrared (FTIR) spectroscopy [53] using a Vertex 70 FTIR-spectrometer (Bruker Optics Inc.) at the Institute of Geological Sciences at the University of Bern (CH). The FTIR spectra have been independently calibrated based on FTIRS analyses of artificial sand/opal mixtures [54] . Opal concentrations determined by means of FTIR spectroscopy show excellent agreement with conventional photometric-based [55] opal concentration determinations ( R 2 =0.91; Supplementary Fig. 4 ) that have been performed on one quarter of the total number of samples ( N =101). However, an increasing offset between photometric and FTIR-based opal measurements towards increasing opal values ( Supplementary Fig. 4 ) might point at incomplete alkaline opal dilution during photometric measurements [55] , potentially caused by a significant fraction of radiolarian skeletons in MD07-3076Q sediments [56] . Opal fluxes have been determined by normalizing the opal data with measured 230 Th concentrations [57] . For these analyses, U- and Th- isotopes were analysed by means of ICP–quadrupole mass spectrometry (iCAP-Q ICP-MS, ThermoFisher) at the Institute for Environmental Physics in Heidelberg, Germany. The contribution of detrital 230 Th has been estimated by assuming a 238 U/ 232 Th ratio of 0.6 and a correction [58] for the detrital 234 U/ 238 U not in secular equilibrium of 0.96. The quality of the analyses and the sample digestion and purification process has been monitored by blanks, certified UREM-11 standard material and replicate measurements of samples. Full replicates ( N =5) yielded an average uncertainty of 2.8 % (two-sigma) of the excess 230 Th concentrations ( Supplementary Table 1 ). The chosen parameter set for the measurements of marine sediments applied here for the first time using an iCAP-Q ICP-MS ( Supplementary Tables 1 and 2 ) puts emphasis on time efficiency for high-matrix sample analyses. Radiocarbon measurements The previously published set of foraminiferal 14 C dates in sediment core MD07-3076Q (ref. 14 ) has been extended by additional paired 14 C measurements of mixed benthic and mono-specific planktonic foraminifera ( N. pachyderma s.). The conventional 14 C ages are reported in Supplementary Tables 3 and 4 . The mean 14 C age uncertainty of the new 14 C data set amounts to 650±270 14 C years ( Supplementary Table 3 ). Foraminifer samples had a mean weight of 5.1±1.0 mg, and weighed always more than 3.4 mg. They have been gently cleaned in methanol, and were subsequently transferred to sealed septum vials after they were completely dry. After evacuation 0.5 ml dry phosphoric acid has been injected into the vials. The acid-carbonate reaction has been sustained for at least 0.5 h at 60 °C. The CO 2 samples were graphitized in the Godwin Radiocarbon Laboratory at the University of Cambridge (UK), along with standards and radiocarbon-dead spar calcite (backgrounds), following a standard hydrogen/iron catalyst protocol [59] . Pressed graphite targets were subsequently analysed by AMS at the 14 Chrono Centre, University of Belfast (UK). Measured 14 C ages have been corrected for mass-dependent fractionation (normalization to δ 13 C=−25‰) and the background radiocarbon content by analysing radiocarbon-dead spar calcite with each sample batch. Paired planktonic and benthic samples have been measured in the same AMS sample carousel. Four paired measurements have resulted in younger benthic than planktonic foraminifera ( Supplementary Fig. 5 ). We have omitted these data from the initial analyses, but including these samples does not alter the general trend of the data ( Supplementary Fig. 5 ). Correlation of marine proxy records with CO 2,atm variations To calculate correlation coefficients R 2 between CO 2,atm variations and 14 C-based deep sub-Antarctic ventilation ages during the last glacial period, that is, 41-22 kyr BP ( Supplementary Fig. 5e ), we interpolated the mean CO 2,atm record [19] at the sampling resolution of the 14 C proxy data. Similarly, the mean CO 2,atm has been interpolated at the resolution of the mean U/Mn c - and the Δδ 13 C-based [O 2 ] records in order to estimate the correlation ( R 2 ) between changes in bottom-water oxygenation and 14 C ventilation in the deep sub-Antarctic Atlantic ( Supplementary Fig. 5f,g ). For these calculations, the mean U/Mn c has been obtained by averaging G. bulloides and Uvigerina spp. U/Mn c (stippled line in Supplementary Fig. 2a ) and the Δδ 13 C-derived [O 2 ] record is based on a 500 year-running average (solid line in Fig. 2f ). Chronostratigraphy of other sub-Antarctic Atlantic cores The most recent age model of sediment core PS2498-1 has been established based on an alignment of variations in lithogenic fluxes with the EPICA Dome C dust record [9] . Because sediment cores MD07-3076Q and PS2498-1 are in close proximity ( Fig. 1 ), we have compared the magnetic susceptibility records and noticed stratigraphic offsets of ±900 years. To allow a faithful inter-core comparison, we have adjusted the chronology of PS2498-1 by aligning the magnetic susceptibility record of PS2498-1 (ref. 60 ) to the magnetic susceptibility record of MD07-3076Q, which has been measured with the GEOTEK Multi-Sensor-Core-Logger aboard R/V Marion Dufresne using a low field susceptibility (Bartington) sensor. For TN057-21, we rely on the most recently established chronology of ref. 28 , which is based on the GICC05 age scale [61] that is equivalent to the AICC2012 age scale used in this study within decades to few hundred years [62] . How to cite this article: Gottschalk, J. et al . Biological and physical controls in the Southern Ocean on past millennial-scale atmospheric CO 2 changes. Nat. Commun. 7:11539 doi: 10.1038/ncomms11539 (2016).